IRF8 inhibits C/EBPα activity to restrain mononuclear phagocyte progenitors from differentiating into neutrophils Myeloid progenitors lose their potential to generate neutrophils when they adopt the mononuclear phagocyte lineage. The mechanism underlying this lineage restriction remains unknown. We here report that the protein expression of IRF8, an essential transcription factor for the development of dendritic cells (DCs) and monocytes, sharply increases at the monocyte-DC progenitor (MDP) stage and remains high in common monocyte progenitors (cMoPs). Irf8 −/− MDPs and cMoPs accumulate but fail to efficiently generate their downstream populations, instead giving rise to neutrophils in vivo . IRF8 physically interacts with the transcription factor C/EBPα and prevents its binding to chromatin in MDPs and cMoPs, blocking the ability of C/EBPα to stimulate transcription and neutrophil differentiation. A partial inhibition of C/EBP activity in Irf8 −/− haematopoietic progenitors alleviates the neutrophil overproduction in vivo . Thus, IRF8 not only bestows monocyte and DC differentiation potential upon mononuclear phagocyte progenitors but also restrains these progenitors from differentiating into neutrophils. Haematopoietic stem cells (HSCs) in the bone marrow self-renew and ultimately differentiate into all types of mature blood and immune cells via several intermediate progenitor stages [1] , [2] . In these processes, intermediate progenitors progress to subsequent stages at the expense of a gradual loss of multi- or oligo-potency. During myelopoiesis, common myeloid progenitors (CMPs) and granulocyte–monocyte progenitors (GMPs) lose their ability to generate neutrophils as they progress to monocyte-dendritic cell (DC) progenitors (MDPs) [3] that give rise to mononuclear phagocytes, that is, monocytes, macrophages and DCs. However, the mechanism by which this lineage restriction occurs is unknown. Cell differentiation requires dynamic changes in gene expression patterns, and these are tightly regulated by cell type-specific transcription factors. The interplay between such transcription factors is important not only to stimulate the differentiation of certain cell lineages but also to inhibit that of other lineages [4] . Defects in these processes in haematopoiesis can result in immunological or haematological disorders such as immunodeficiency and leukaemias [5] . Interferon regulatory factor-8 (IRF8) is a haematopoietic cell-specific member of the IRF transcription factor family. Irf8 −/− mice develop immunodeficiency and a chronic myeloid leukaemia-like syndrome [6] , [7] . Subsequent studies revealed that IRF8 regulates the development of multiple immune cell types [8] . IRF8 is required for the generation of mouse monocytes (particularly Ly6C + monocytes) [9] , [10] , classical DCs (cDCs; particularly CD8α + DCs) and plasmacytoid DCs (pDCs) [11] , [12] , [13] that express high levels of IRF8 (refs 14 , 15 ). At the progenitor level, Irf8 −/− mice harbour increased numbers of GMPs and MDPs but lack common DC progenitors (CDPs) [16] , [17] . Recent studies have suggested that Irf8 transcript expression is relatively high in MDPs, CDPs and common monocyte progenitors (cMoPs) [18] , [19] , [20] . Importantly, mutations in the human IRF8 gene are associated with DC and monocyte deficiency [21] . On the other hand, IRF8 deficiencies cause severe neutrophilia in mice and humans [6] , [21] . As a possible explanation for this phenotype, we have previously demonstrated that IRF8 strongly inhibits growth and neutrophil differentiation of granulocyte colony-stimulating factor (G-CSF)-treated myeloid progenitors [10] , [22] . Of note, neutrophils do not express Irf8 (refs 15 , 18 ), suggesting that IRF8 may act at progenitor stages to inhibit this lineage. However, the exact differentiation stage at which IRF8 inhibits neutrophil differentiation remains elusive. IRF8 binds to specific DNA sequences only when it forms heterodimers with partner transcription factors. The IRF8–PU.1 heterodimer transcriptionally activates genes containing the ETS-IRF composite element (EICE) or the IRF-ETS composite sequence (IECS) [8] , [9] . Since PU.1 is essential for the development of myeloid cells, particularly monocytes and DCs, PU.1 is undoubtedly a critical partner of IRF8 in promoting their differentiation. In addition, the IRF8–BATF heterodimer binds to the activating protein-1-IRF composite element to promote gene activation during DC differentiation [23] . It has been reported in overexpression experiments that IRF8 also acts as a transcriptional repressor when it binds to the interferon-stimulated response element in association with IRF1 or IRF2 (ref. 24 ). However, our recent analysis of genome-wide IRF8 behaviour in myeloid progenitors has suggested that IRF8, as a DNA binding protein, mainly functions as an activator in association with PU.1, inducing a chromatin signature of enhancers (that is, histone H3 lysine 4 monomethylation) when promoting monocyte differentiation [9] . In contrast to the well-studied mode of action of IRF8 in stimulating differentiation, nothing is yet known regarding the molecular mechanism by which IRF8 inhibits neutrophil differentiation. In our current study, we found that IRF8 expression is sharply increased at the MDP stage and is essential in vivo for restraining MDPs and cMoPs from developing into neutrophils. We further demonstrate that IRF8 physically interacts with and inhibits the transcriptional activity of CCAAT/enhancer-binding protein α (C/EBPα), a transcription factor that strongly induces neutrophil differentiation. A partial inhibition of C/EBP activity in Irf8 −/− haematopoietic progenitors alleviates the overproduction of neutrophils in vivo . These results clarified how and the stage at which IRF8 inhibits neutrophil differentiation, thus shedding light on the mechanism underlying the commitment of the mononuclear phagocyte lineage. IRF8 protein expression in myeloid progenitor populations We examined IRF8 expression in bone marrow myeloid progenitor cell populations on a per cell basis using intracellular immunostaining followed by flow cytometry (see Supplementary Fig. 1 for antibody validation). IRF8 protein was found to be highly expressed in MDPs ( Fig. 1a ). MDPs were originally identified as myeloid progenitor cells expressing CD117 and a Cx3cr1 promoter-driven GFP ( Cx3cr1 -GFP) [25] reporter, and subsequently described as a CD115 + myeloid progenitor population [26] . More than 80% of ‘ Cx3cr1 -GFP + ’ MDPs and essentially all ‘CD115 + ’ MDPs expressed high levels of IRF8. Subpopulations of CMPs and GMPs also expressed graded levels of IRF8 that closely correlated with that of CD115 ( Fig. 1b ). This suggests that these subpopulations are becoming or are already MDPs, which is consistent with the fact that significant portions of CMPs and GMPs overlap with MDPs [25] , [26] . The HSC-enriched population (lineage markers-negative (Lin − ) Sca-1 + c-Kit/CD117 + ; LSK) barely expressed IRF8 ( Fig. 1c ). Hence, IRF8 expression in LSK cells and CD115 − early myeloid progenitors (MPs) is low or absent, but sharply increases when they differentiate to MDPs. IRF8 expression continued to be high in CDPs ( Fig. 1d ). CD115 − CDPs and cMoPs, recently identified as additional populations with prominent pDC and monocyte differentiation potentials, respectively [20] , [27] , also highly expressed IRF8 protein ( Fig. 1d,e ). 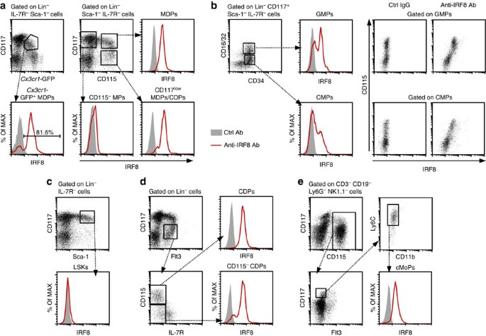Figure 1: Mononuclear phagocyte progenitors express high levels of IRF8 protein. (a–e) IRF8 protein expression in bone marrow progenitor populations was examined by immunostaining followed by flow cytometry. Bone marrow progenitors were defined as follows:Cx3cr1-GFP+MDPs, Lin−IL-7R−Sca-1−CD117+Cx3cr1-GFP+(a); MDPs, Lin−IL-7R−Sca-1−CD117+CD115+(a); CD115−MPs, Lin−IL-7R−Sca-1−CD117+CD115−(a); CD117lowMDPs/CDPs, Lin−IL-7R−Sca-1−CD117lowCD115+(a); GMPs, Lin−IL-7R−Sca-1−CD117+CD34+CD16/32+(b); CMPs, Lin−IL-7R−Sca-1−CD117+CD34+CD16/32low(b); LSKs, Lin−IL-7R−Sca-1+CD117+(c); CDPs, Lin−IL-7R−CD117lowCD115+Flt3+(d); CD115−CDPs, Lin−IL-7R−CD117lowCD115−Flt3+(d); cMoPs, CD3−CD19−Ly6G−NK1.1−CD117+CD115+Flt3−cells (e). Histograms indicate anti-IRF8 antibody (Ab; red) and control (Ctrl) Ab (grey shaded) staining. Similar results were obtained from four independent experiments. Figure 1: Mononuclear phagocyte progenitors express high levels of IRF8 protein. ( a – e ) IRF8 protein expression in bone marrow progenitor populations was examined by immunostaining followed by flow cytometry. Bone marrow progenitors were defined as follows: Cx3cr1 -GFP + MDPs, Lin − IL-7R − Sca-1 − CD117 + Cx3cr1-GFP + ( a ); MDPs, Lin − IL-7R − Sca-1 − CD117 + CD115 + ( a ); CD115 − MPs, Lin − IL-7R − Sca-1 − CD117 + CD115 − ( a ); CD117 low MDPs/CDPs, Lin − IL-7R − Sca-1 − CD117 low CD115 + ( a ); GMPs, Lin − IL-7R − Sca-1 − CD117 + CD34 + CD16/32 + ( b ); CMPs, Lin − IL-7R − Sca-1 − CD117 + CD34 + CD16/32 low ( b ); LSKs, Lin − IL-7R − Sca-1 + CD117 + ( c ); CDPs, Lin − IL-7R − CD117 low CD115 + Flt3 + ( d ); CD115 − CDPs, Lin − IL-7R − CD117 low CD115 − Flt3 + ( d ); cMoPs, CD3 − CD19 − Ly6G − NK1.1 − CD117 + CD115 + Flt3 − cells ( e ). Histograms indicate anti-IRF8 antibody (Ab; red) and control (Ctrl) Ab (grey shaded) staining. Similar results were obtained from four independent experiments. Full size image Irf8 −/− MDPs and cMoPs aberrantly give rise to neutrophils Comprehensive analysis comparing wild-type (WT) and Irf8 −/− myeloid progenitor populations is shown in Fig. 2 . We confirmed previously reported findings [18] that Irf8 −/− myeloid progenitors accumulate in MDPs and lack CD117 low MDPs/CDPs [26] ( Fig. 2a,b ). We refer to the CD117 low MDP population as CD117 low MDPs/CDPs because most CDPs reside in the CD117 low MDP population, yet CD117 low MDPs still produce some macrophages [26] . Irf8 −/− MDPs were found to express another MDP marker, Cx3cr1 -GFP, suggesting that they are bona fide MDPs ( Supplementary Fig. 2 ). We observed that the numbers of CD115 − CDPs and pre-cDCs (committed cDC precursors) were also severely diminished in Irf8 −/− mice ( Fig. 2b,c ). Furthermore, we found that Irf8 −/− mice accumulate cMoPs (6.9-fold compared with WT cMoPs) to an even greater extent than MDPs (3.6-fold compared with WT MDPs), and, as we have reported previously [9] , lack Ly6C + monocytes ( Fig. 2d ). These data suggest that the differentiation arrest in Irf8 −/− mice occurs at the transition from MDPs to CD117 low MDPs/CDPs and from cMoPs to Ly6C + monocytes. 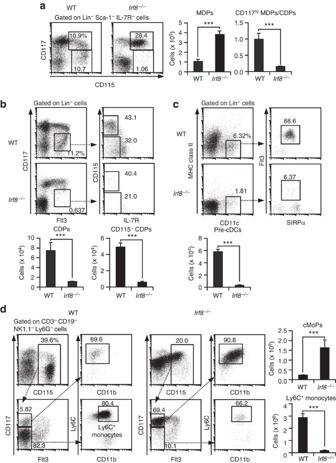Figure 2:Irf8−/−mice have increased MDP and cMoP counts but lack CDPs and Ly6C+monocytes. (a–d) Bone marrow cells from WT andIrf8−/−mice were analysed for myeloid progenitors and Ly6C+monocytes by flow cytometry. The cell numbers of each population per lower mouse limb were calculated. Values are the mean±s.d. from three or four mice. ***P<0.001 (Student’st-test). Similar results were obtained from four independent experiments in total. Figure 2: Irf8 −/− mice have increased MDP and cMoP counts but lack CDPs and Ly6C + monocytes. ( a – d ) Bone marrow cells from WT and Irf8 −/− mice were analysed for myeloid progenitors and Ly6C + monocytes by flow cytometry. The cell numbers of each population per lower mouse limb were calculated. Values are the mean±s.d. from three or four mice. *** P <0.001 (Student’s t -test). Similar results were obtained from four independent experiments in total. Full size image The fate of Irf8 −/− MDPs and cMoPs then became a key question. To answer this question, we isolated CD117 + MDPs and cMoPs from WT and Irf8 −/− mice and then transplanted these cells into lethally irradiated mice (1.0 × 10 4 cells per mouse). As expected, WT MDPs generated monocytes (mostly Ly6C + ) in the bone marrow and cDCs in the spleen ( Fig. 3a ). MDP-derived pDCs were not detectable under our experimental conditions, consistent with a previous report [25] . On the other hand, Irf8 −/− MDPs failed to efficiently yield bone marrow monocytes and splenic cDCs, especially the CD8α + subset, but, intriguingly, instead gave rise to a large number of neutrophils. In mice transplanted with WT MDPs, almost no neutrophils could be detected (only 0.064 × 10 4 and 0.058 × 10 4 neutrophils in the lower limb bones and spleen on average, respectively). However, in mice transplanted with Irf8 −/− MDPs, we could detect an average of 3.2 × 10 4 and 7.1 × 10 4 neutrophils in the lower limb bones (a 50-fold increase) and spleen (a 121-fold increase), respectively. Moreover, Irf8 −/− cMoPs failed to efficiently produce monocytes and, again, aberrantly gave rise to a large number of neutrophils ( Fig. 3b ). Thus, many Irf8 −/− MDPs may pass through cMoPs to produce neutrophils, although it is also possible that some Irf8 −/− MDPs directly differentiate into neutrophils. We also cultured MDPs in vitro in the presence of stem cell factor (SCF), macrophage colony-stimulating factor (M-CSF), FMS-like tyrosine kinase 3 ligand (Flt3L) and G-CSF. We found that ~50% of the cells generated from Irf8 −/− MDPs, but only 3% of those derived from WT MDPs, were neutrophils ( Fig. 3c ). These results suggest that IRF8 is essential not only to bestow monocyte and DC differentiation potential upon MDPs and cMoPs, respectively, but also to restrain these populations from differentiating into neutrophils. 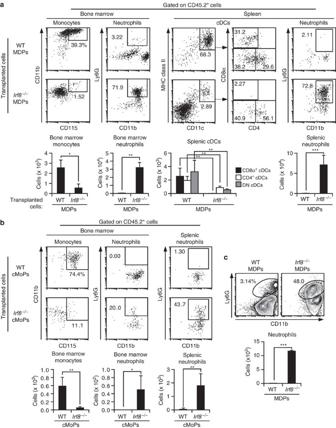Figure 3:Irf8−/−MDPs and cMoPs aberrantly produce a large number of neutrophils. (a,b) Flow cytometric analysis of bone marrow monocytes, splenic cDCs and splenic neutrophils 5 and 2 days after intravenous transplantation of MDPs (a) and cMoPs (b), respectively. Ten thousand progenitor cells from WT orIrf8−/−mice (CD45.2+) were transplanted into irradiated Ly5.1 mice (CD45.2−), and donor-derived (CD45.2+) cells were analysed. Bone marrow CD117+cells were gated out to exclude progenitor cells. Absolute cell numbers (per spleen or lower limbs of a mouse) of the indicated progeny cells derived from transplanted MDPs and cMoPs are shown in the bar graphs. Values are the mean±s.d. from three or four mice. Similar results were obtained from three independent experiments. (c) Five thousand MDPs were cultured for 7 days in the presence of SCF, M-CSF, Flt3L and G-CSF. Neutrophils derived from these MDPs were analysed by flow cytometry. Values in the bar graph are the mean±s.d. of triplicate determinations. Similar results were obtained from three independent experiments. *P<0.05, **P<0.01, ***P<0.001 (Student’st-test). Figure 3: Irf8 −/− MDPs and cMoPs aberrantly produce a large number of neutrophils. ( a , b ) Flow cytometric analysis of bone marrow monocytes, splenic cDCs and splenic neutrophils 5 and 2 days after intravenous transplantation of MDPs ( a ) and cMoPs ( b ), respectively. Ten thousand progenitor cells from WT or Irf8 −/− mice (CD45.2 + ) were transplanted into irradiated Ly5.1 mice (CD45.2 − ), and donor-derived (CD45.2 + ) cells were analysed. Bone marrow CD117 + cells were gated out to exclude progenitor cells. Absolute cell numbers (per spleen or lower limbs of a mouse) of the indicated progeny cells derived from transplanted MDPs and cMoPs are shown in the bar graphs. Values are the mean±s.d. from three or four mice. Similar results were obtained from three independent experiments. ( c ) Five thousand MDPs were cultured for 7 days in the presence of SCF, M-CSF, Flt3L and G-CSF. Neutrophils derived from these MDPs were analysed by flow cytometry. Values in the bar graph are the mean±s.d. of triplicate determinations. Similar results were obtained from three independent experiments. * P <0.05, ** P <0.01, *** P <0.001 (Student’s t -test). Full size image Transcriptome analysis of MDPs and cMoPs in Irf8 −/− mice To investigate the mechanism by which IRF8 inhibits neutrophil differentiation, we performed transcriptome analysis by microarray of MDPs and cMoPs in WT and Irf8 −/− mice (the quality control for the microarray data is shown in Supplementary Fig. 3 ). Although it is reasonable to speculate that the loss of IRF8 results in the upregulation of genes critical for neutrophil differentiation, given the results of our previous genome-wide analysis on the behaviour of IRF8 in myeloid progenitors [9] , it seemed unlikely that IRF8 directly acts as a transcriptional repressor. To predict the transcription factor(s) responsible for the aberrant production of neutrophils from Irf8 −/− MDPs and cMoPs, we used Ingenuity Pathway Analysis (IPA) software. In both MDPs and cMoPs, C/EBPs were identified by IPA as candidate transcription factors activated in the absence of IRF8 ( Supplementary Fig. 3c,d ). Examples of known C/EBP target genes with significantly higher expression in Irf8 −/− than WT progenitors included Mmp8 , S100a8 and Hsd11b1 ( Supplementary Fig. 4a ). Among the C/EBPs, C/EBPα and C/EBPε have been extensively shown to be capable of driving myeloid progenitor cell differentiation into neutrophils [4] , [5] . Despite the upregulation of C/EBP target genes, neither the expression of Cebpa nor Cebpe per se was found to be drastically upregulated in Irf8 −/− MDPs ( Supplementary Fig. 4a ), suggesting that IRF8 may regulate the activity, rather than the expression levels, of the C/EBP(s). In Irf8 −/− cMoPs, Cebpe expression was increased compared with that in WT cMoPs by 3.45-fold, presumably because Cepbe is a target gene of C/EBPα. Consistent with these transcript levels, the expression of C/EBPα protein was comparable in Irf8 −/− MDPs and only modestly elevated in cMoPs compared with WT counterparts ( Supplementary Fig. 4b ). Hence, we focused on C/EBPα in our subsequent experiments. We note here that NF-κB was also identified as a transcription factor complex activated in Irf8 −/− MDPs and cMoPs, and this may warrant future investigation, especially in terms of the regulation of apoptosis by IRF8. IRF8 inhibits transcriptional activation by C/EBPα To examine the effects of IRF8 on C/EBPα-dependent transcriptional activation, we first performed a reporter assay. We transduced 293T cells with a reporter lentivirus harbouring four copies of the C/EBP response element, followed by a minimal cytomegalovirus (CMV) promoter and cDNA insert encoding GFP (GreenFire1-C/EBPα). These reporter cells were then transfected with expression plasmids for C/EBPα and IRF8. C/EBPα strongly activated the reporter and IRF8 inhibited this activation in a dose-dependent manner ( Supplementary Fig. 5 ). We next tested IRF8 K79E and IRF8 R289E , which have a mutation in the DNA binding domain (DBD) and IRF association domain, respectively. IRF8 K79E is defective in DNA binding, while IRF8 R289E cannot interact with PU.1 and other IRFs [28] . Neither mutant is capable of inducing macrophage and DC differentiation [10] , [28] , [29] . Interestingly, IRF8 R289E still blocked the transactivation by C/EBPα, whereas IRF8 K79E lost this inhibitory effect, suggesting the involvement of DBD in the inhibition of C/EBPα activity. IRF8 did not downregulate the expression of exogenous C/EBPα (see immunoblotting analysis in the section following the next). IRF8 inhibits C/EBPα-induced neutrophil differentiation To investigate whether IRF8 has indeed any antagonistic effects on C/EBPα in neutrophil differentiation, we used the 32Dcl.3 myeloid progenitor cell line that has been shown to differentiate into neutrophils upon the exogenous expression of C/EBPα [30] , [31] . 32Dcl.3 cells were retrovirally transduced with IRF8 and/or C/EBPα, and their morphology was monitored. When transduced with C/EBPα alone, 40% of these cells exhibited typical neutrophil features such as segmented nuclei by day 4 ( Fig. 4a ). IRF8 alone did not affect cell morphology as previously reported [10] . However, when IRF8 was coexpressed, only 12% of the cells displayed a neutrophil-like morphology and some displayed cytoplasmic vacuoles that are a feature of monocytes. The expression level of C/EBPα protein was found not to be downregulated by IRF8 ( Fig. 4b ). These results indicate that IRF8 is capable of inhibiting C/EBPα-induced neutrophil differentiation. 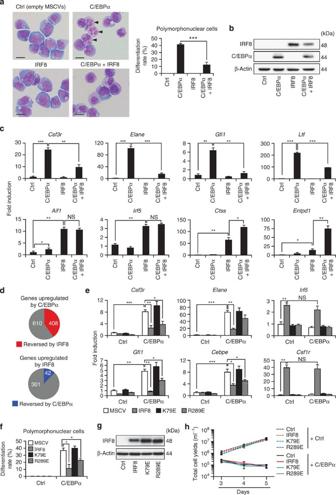Figure 4: IRF8 inhibits C/EBPα-induced neutrophil differentiation. (a) Wright–Giemsa staining (left; original magnification, × 600) and polymorphonuclear cell frequencies (right bar graph). 32Dcl.3 cells were transduced with empty MSCV-CD8t or MSCV-IRF8-CD8t and then with empty MSCV-puro or MSCV-C/EBPα-puro retroviruses. Cells were analysed 4 days post-C/EBPα transduction. Arrowheads indicate typical polymorphonuclear cells. Bars, 10 μm. Values in the bar graph are the mean±s.d. from five independent experiments. ***P<0.001 (Student’st-test). (b) Immunoblotting of C/EBPα and IRF8 in transduced 32Dcl.3 cells on day 3. (c) Expression of C/EBPα- or IRF8-inducible genes in 32Dcl.3 cells transduced with C/EBPα and/or IRF8. Transcript levels were analysed 3 days post-C/EBPα transduction by RT–qPCR using the ΔΔCT method. Data were normalized to theGapdhlevels, and the values shown are relative to those in empty vector-transduced cells (mean±s.d. from three independent experiments). *P<0.05, **P<0.01, ***P<0.001 (Student’st-test). (d) Pie charts for the numbers of genes that displayed a more than threefold increase in expression induced by C/EBPα (upper panel) and IRF8 (lower panel), and those reversed by IRF8 (red) and C/EBPα (blue), respectively. (e) Expression of C/EBPα- or IRF8-inducible genes in 32Dcl.3 cells transduced with C/EBPα and/or IRF8 mutants. Transcript levels were analysed 3 days post-C/EBPα transduction by RT–qPCR. *P<0.05, **P<0.01, ***P<0.001 (Student’st-test). (f) Polymorphonuclear cell frequencies in 32Dcl.3 cells transduced with C/EBPα and/or IRF8 (WT or mutants) examined by Wright–Giemsa staining. Values in the bar graph are the mean±s.d. from three independent experiments. *P<0.05 (Student’st-test). (g) Immunoblotting analysis of IRF8 mutants. (h) Growth rate analysis. Data are expressed as the mean±s.d. of triplicate determinations. Ctrl, control; NS, not significant. Figure 4: IRF8 inhibits C/EBPα-induced neutrophil differentiation. ( a ) Wright–Giemsa staining (left; original magnification, × 600) and polymorphonuclear cell frequencies (right bar graph). 32Dcl.3 cells were transduced with empty MSCV-CD8t or MSCV-IRF8-CD8t and then with empty MSCV-puro or MSCV-C/EBPα-puro retroviruses. Cells were analysed 4 days post-C/EBPα transduction. Arrowheads indicate typical polymorphonuclear cells. Bars, 10 μm. Values in the bar graph are the mean±s.d. from five independent experiments. *** P <0.001 (Student’s t -test). ( b ) Immunoblotting of C/EBPα and IRF8 in transduced 32Dcl.3 cells on day 3. ( c ) Expression of C/EBPα- or IRF8-inducible genes in 32Dcl.3 cells transduced with C/EBPα and/or IRF8. Transcript levels were analysed 3 days post-C/EBPα transduction by RT–qPCR using the ΔΔCT method. Data were normalized to the Gapdh levels, and the values shown are relative to those in empty vector-transduced cells (mean±s.d. from three independent experiments). * P <0.05, ** P <0.01, *** P <0.001 (Student’s t -test). ( d ) Pie charts for the numbers of genes that displayed a more than threefold increase in expression induced by C/EBPα (upper panel) and IRF8 (lower panel), and those reversed by IRF8 (red) and C/EBPα (blue), respectively. ( e ) Expression of C/EBPα- or IRF8-inducible genes in 32Dcl.3 cells transduced with C/EBPα and/or IRF8 mutants. Transcript levels were analysed 3 days post-C/EBPα transduction by RT–qPCR. * P <0.05, ** P <0.01, *** P <0.001 (Student’s t -test). ( f ) Polymorphonuclear cell frequencies in 32Dcl.3 cells transduced with C/EBPα and/or IRF8 (WT or mutants) examined by Wright–Giemsa staining. Values in the bar graph are the mean±s.d. from three independent experiments. * P <0.05 (Student’s t -test). ( g ) Immunoblotting analysis of IRF8 mutants. ( h ) Growth rate analysis. Data are expressed as the mean±s.d. of triplicate determinations. Ctrl, control; NS, not significant. Full size image We next performed quantitative PCR with reverse transcription (RT–qPCR) to analyse the expression of target genes of C/EBPα and IRF8. The C/EBPα target genes such as Csf3r , Elane , Gfi1 and Ltf were markedly suppressed by IRF8 transduction. On the other hand, the induction of IRF8 target genes such as Aif1 , Irf5 , Ctss and Entpd1 was not suppressed by C/EBPα ( Fig. 4c ). Transcriptome analysis by microarray ( Fig. 4d ) revealed that among the 1,018 genes upregulated by C/EBPα (fold change (FC)>3 and false discovery rate (FDR) <0.05), the expression of 408 genes (40.1%) was suppressed by coexpression of IRF8 (FC <0.5 and FDR <0.05). On the other hand, among the 343 IRF8-upregulated genes (FC >3 and FDR <0.05), the expression of only 42 genes (12.2%) was suppressed by coexpression of C/EBPα (FC <0.5 and FDR<0.05). We also found that IRF8 R289E but not IRF8 K79E suppressed target gene induction and neutrophil differentiation by C/EBPα ( Fig. 4e–g ), which is consistent with the results in 293T cells. Of note, neither IRF8 K79E nor IRF8 R289E induces monocyte differentiation-related IRF8 target genes [22] , [29] , suggesting that the modes of IRF8 action in promoting monocyte differentiation and inhibiting neutrophil differentiation are indeed distinct. Cell growth was found to be markedly inhibited by C/EBPα as expected from previous findings [32] , [33] ( Fig. 4h ). IRF8 alone had no impact on cell growth in 32Dcl.3 cells as also previously reported [10] . Interestingly, despite the fact that IRF8 and IRF8 R289E inhibited neutrophil differentiation in our current analysis, neither of them affected the growth arrest induced by C/EBPα ( Fig. 4h ; see Discussion section). IRF8 physically interacts with C/EBPα To clarify the mechanism by which IRF8 inhibits C/EBPα activity, we examined whether these factors physically interact. By using 293T cells transfected with IRF8 and C/EBPα, we found that IRF8 co-immunoprecipitated C/EBPα ( Fig. 5a ). Interestingly, IRF8 R289E but not IRF8 K79E also co-immunoprecipitated C/EBPα, which is congruent with our reporter assay data. These results suggest that IRF8, via its DBD, physically interacts with C/EBPα to inhibit its activity. The interaction between IRF8 and C/EBPα was also detected by an amplified luminescence proximity homogeneous assay screen (AlphaScreen) using recombinant IRF8 and C/EBPα generated by the wheat-germ cell-free protein production system ( Fig. 5b ), suggesting that this interaction is direct. 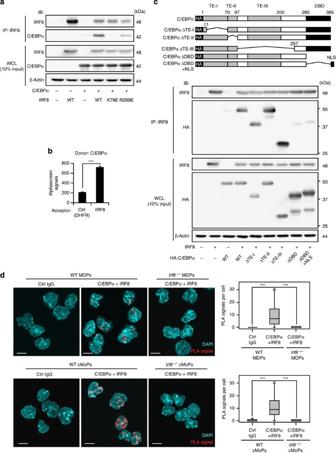Figure 5: Direct interaction between IRF8 and C/EBPα. (a) Co-immunoprecipitation of C/EBPα and IRF8, IRF8K79Eor IRF8R289Ein 293T cells. IP, immunoprecipitation; WCL, whole-cell lysate; IB, immunoblot. (b)In vitrobinding analysis of IRF8 with C/EBPα using AlphaScreen.Escherichia colidihydrofolate reductase (DHFR) was used as a negative control (Ctrl). The emission from the acceptor beads was measured and is shown as AlphaScreen signals. All values are the mean±s.d. from three independent reactions. ***P<0.001 (Student’st-test). (c) Co-immunoprecipitation of IRF8 and C/EBPα or its deletion mutants. Diagrams of C/EBPα and its mutants are shown on the top. The results are representative of three independent experiments. (d)In situPLA in purified MDPs and cMoPs. Interaction between IRF8 and C/EBPα were visualized as punctate fluorescent spots (PLA signals) detected by confocal microscopy. In the box plot, the numbers of PLA spots per cell were counted in 100 cells each. The results are representative of two independent experiments. Scale bars, 10 μm. ***P<0.001 (Student’st-test). Figure 5: Direct interaction between IRF8 and C/EBPα. ( a ) Co-immunoprecipitation of C/EBPα and IRF8, IRF8 K79E or IRF8 R289E in 293T cells. IP, immunoprecipitation; WCL, whole-cell lysate; IB, immunoblot. ( b ) In vitro binding analysis of IRF8 with C/EBPα using AlphaScreen. Escherichia coli dihydrofolate reductase (DHFR) was used as a negative control (Ctrl). The emission from the acceptor beads was measured and is shown as AlphaScreen signals. All values are the mean±s.d. from three independent reactions. *** P <0.001 (Student’s t -test). ( c ) Co-immunoprecipitation of IRF8 and C/EBPα or its deletion mutants. Diagrams of C/EBPα and its mutants are shown on the top. The results are representative of three independent experiments. ( d ) In situ PLA in purified MDPs and cMoPs. Interaction between IRF8 and C/EBPα were visualized as punctate fluorescent spots (PLA signals) detected by confocal microscopy. In the box plot, the numbers of PLA spots per cell were counted in 100 cells each. The results are representative of two independent experiments. Scale bars, 10 μm. *** P <0.001 (Student’s t -test). Full size image To identify the domain of C/EBPα that is required for the interaction with IRF8, we constructed mutant forms of C/EBPα. These included deletion mutants of the transactivation element-I (ΔTE-I), ΔTE-II, ΔTE-III and of the DBD (ΔDBD) ( Fig. 5c ). Because the DBD contains a region required for nuclear entry, we also constructed a mutant in which a nuclear localization signal (NLS) was combined with the DBD deletion (ΔDBD+NLS). The subcellular localization of C/EBPα mutants was validated by imaging of yellow fluorescent protein (YFP) signals in 293T cells transfected with YFP-C/EBPα chimeras ( Supplementary Fig. 6 ). Using 293T cells transfected with IRF8 and the C/EBPα mutants, we found that IRF8 co-immunoprecipitated the ΔTE-I, ΔTE-II and ΔTE-III mutants, but not the ΔDBD and ΔDBD+NLS products ( Fig. 5c ). These results indicate that IRF8 and C/EBPα interact with each other through their DBDs. The DBD of C/EBPα is subdivided into a basic region (BR) and leucine zipper (LZ) that are necessary for DNA binding and dimerization, respectively [34] . We also constructed ΔBR and ΔLZ mutants combined with an NLS ( Supplementary Fig. 7a,b ), which we cotransfected with IRF8. Both of the ΔBR and ΔLZ mutants could be co-immunoprecipitated by IRF8, suggesting that each of these regions can independently interact with IRF8 ( Supplementary Fig. 7c ). We further examined whether such interactions would occur between endogenous proteins in MDPs and cMoPs. To this end, we performed an in situ proximity ligation assay (PLA) in purified MDPs and cMoPs. Multiple strong signals were observed, indicating the association between endogenous IRF8 and C/EBPα in WT MDPs and cMoPs ( Fig. 5d ). As a further endorsement of the specificity of these signals, essentially no PLA signals between IRF8 and C/EBPα were observed in Irf8 −/− MDPs and cMoPs. IRF8 prevents C/EBPα from binding to chromatin The above findings that DBDs are involved in the interaction between IRF8 and C/EBPα prompted us to examine the chromatin binding of these proteins. We performed a chromatin immunoprecipitation (ChIP)–qPCR assay using anti-C/EBPα and anti-IRF8 antibodies in 32Dcl.3 cells transduced with IRF8 and/or C/EBPα. ChIP signals for C/EBPα on the promoters of C/EBPα target genes Csf3r , Elane and Ltf were significantly suppressed by IRF8 ( Fig. 6a ). On the other hand, ChIP signals of IRF8 on the promoters of IRF8 target genes Ctss and Entpd1 were not suppressed by C/EBPα. Both IRF8 and C/EBPα bound to the promoter of Aif1 , which was induced either by IRF8 or C/EBPα. Again, the binding of C/EBPα to this promoter was repressed by IRF8, while that of IRF8 was instead augmented by C/EBPα. These results indicate that IRF8 inhibits chromatin binding by C/EBPα to thereby block neutrophil differentiation, but not the other way around. 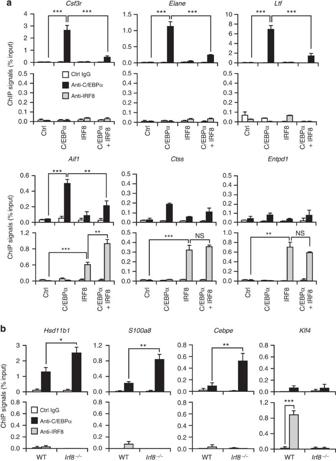Figure 6: IRF8 prevents C/EBPα from binding to chromatin. (a,b) ChIP–qPCR assay using anti-C/EBPα and anti-IRF8 antibodies. (a) 32Dcl.3 cells were transduced with C/EBPα and/or IRF8 as described inFig. 4. Cells were analysed 3 days post-C/EBPα transduction. Values are the mean±s.d. from four independent experiments. (b) CD115+progenitor cells (CD3−CD11b−CD19−Ly6G−NK1.1−CD117+CD115+cells) were freshly isolated and analysed. Values are the mean±s.d. from three independent experiments.*P<0.05, **P<0.01, ***P<0.001 (Student’st-test). Ctrl, control; NS, not significant. Figure 6: IRF8 prevents C/EBPα from binding to chromatin. ( a , b ) ChIP–qPCR assay using anti-C/EBPα and anti-IRF8 antibodies. ( a ) 32Dcl.3 cells were transduced with C/EBPα and/or IRF8 as described in Fig. 4 . Cells were analysed 3 days post-C/EBPα transduction. Values are the mean±s.d. from four independent experiments. ( b ) CD115 + progenitor cells (CD3 − CD11b − CD19 − Ly6G − NK1.1 − CD117 + CD115 + cells) were freshly isolated and analysed. Values are the mean±s.d. from three independent experiments. * P <0.05, ** P <0.01, *** P <0.001 (Student’s t -test). Ctrl, control; NS, not significant. Full size image We further examined whether an IRF8 deficiency causes enhanced binding of C/EBPα to chromatin in vivo . We isolated CD115 + progenitor cells (CD3 − CD11b − CD19 − Ly6G − NK1.1 − CD117 + CD115 + ), which comprised MDPs and cMoPs, from WT and Irf8 −/− bone marrow and performed ChIP–qPCR. The binding of C/EBPα to its target genes Hsd11b1 , S100a8 and Cebpe was significantly augmented in Irf8 −/− CD115 + progenitor cells compared with WT cells ( Fig. 6b ), which is consistent with the increased expression of these genes in Irf8 −/− MDPs or cMoPs ( Supplementary Fig. 4a ). The binding of IRF8 to these C/EBPα target genes in WT CD115 + progenitor cells was at near background levels, while IRF8 strongly bound to its authentic target, the Klf4 enhancer [9] . The ChIP signals for C/EBPα on the IRF8-bound Klf4 enhancer region were relatively low. These in vivo data further support our notion that IRF8 inhibits C/EBPα binding to chromatin to suppress its transcriptional activity. To gain insight into how IRF8 suppresses C/EBPα binding to chromatin, we examined whether IRF8 prevents C/EBPα homodimer formation. FLAG-tagged C/EBPα very efficiently co-immunoprecipitated haemagglutinin (HA)-tagged C/EBPα, which was not inhibited by IRF8 ( Supplementary Fig. 7d ). These results suggest that IRF8 does not inhibit the dimerization of C/EBPα, but probably interacts with the C/EBPα dimer to prevent its binding to chromatin. C/EBP inhibition alleviates neutrophillia in Irf8 −/− mice If the failure to inhibit C/EBPα is a cause of neutrophilia in Irf8 −/− mice, the symptom would be ameliorated by reducing C/EBP activity in vivo . We transduced WT or Irf8 −/− bone marrow progenitor cells with a retrovirus encoding a dominant-negative form of C/EBP (A-C/EBP) along with enhanced GFP (EGFP), and transplanted these cells into irradiated mice. A-C/EBP contains the LZ domain conserved in the C/EBPs but lacks a functional DBD and TEs, forms stable inactive heterodimers with C/EBPs and thus prevents C/EBPs from binding to DNA [35] . GFP-positive (that is, retrovirus-transduced) cells in the spleen were analysed by flow cytometry 4 weeks after transplantation. As expected, engraftment of empty retrovirus-transduced Irf8 −/− cells resulted in a significant increase in neutrophil counts, whereas the generation of Ly6C + monocytes, pDCs and CD8α + DCs was severely impaired compared with empty retrovirus-transduced WT cells ( Fig. 7a,b ). On the other hand, mice transplanted with A-C/EBP-transduced Irf8 −/− progenitor cells clearly showed inhibition of neutrophil overproduction, that is, the neutrophil counts returned to almost normal levels. The generation of Ly6C + monocytes, pDCs and CD8α + DCs was not restored by A-C/EBP. In mice transplanted with A-C/EBP-transduced WT progenitor cells, a mild reduction of neutrophil and monocyte counts and a modest increase in DC counts were observed, consistent with the previously reported functions of C/EBPα [36] . This also suggests that the inhibition of C/EBP activity by A-C/EBP is partial. These results support the notion that the enhancement of C/EBP activity causes an overproduction of neutrophils in the absence of IRF8. 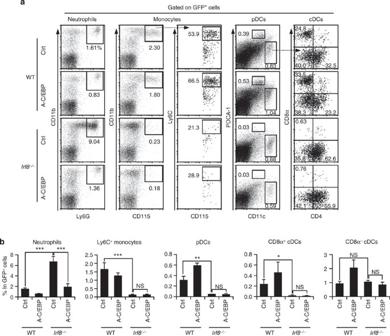Figure 7: A dominant-negative C/EBP remedies the aberrant overproduction of neutrophils fromIrf8−/−haematopoietic progenitors. (a) WT orIrf8−/−Lin−cells were transduced with empty pGCsam-EGFP (Ctrl) or A-C/EBP-EGFP, and transplanted into irradiated WT mice. Retrovirus-transduced (GFP+) cells in the spleen of recipient mice were analysed by flow cytometry at 3 weeks post transplantation. Data are representative of four independent experiments with similar results. (b) The frequencies of the indicated progeny cells in GFP+splenic cell populations. Values are the mean±s.d. from eight mice of each group in four independent experiments. *P<0.05, **P<0.01, ***P<0.001 (Student’st-test). NS, not significant. Figure 7: A dominant-negative C/EBP remedies the aberrant overproduction of neutrophils from Irf8 −/− haematopoietic progenitors. ( a ) WT or Irf8 −/− Lin − cells were transduced with empty pGCsam-EGFP (Ctrl) or A-C/EBP-EGFP, and transplanted into irradiated WT mice. Retrovirus-transduced (GFP + ) cells in the spleen of recipient mice were analysed by flow cytometry at 3 weeks post transplantation. Data are representative of four independent experiments with similar results. ( b ) The frequencies of the indicated progeny cells in GFP + splenic cell populations. Values are the mean±s.d. from eight mice of each group in four independent experiments. * P <0.05, ** P <0.01, *** P <0.001 (Student’s t -test). NS, not significant. Full size image Our current findings have unveiled a molecular mechanism that regulates the differentiation potential of MDPs and cMoPs. We pinpointed MDPs as the stage at which IRF8 expression becomes high. IRF8 is essential not only for MDP and cMoP progression to CD117 low MDPs/CDPs and Ly6C + monocytes, respectively, but also for preventing these progenitors from developing into neutrophils. We show from our present data that IRF8 interacts with C/EBPα in MDPs and cMoPs, interferes with the ability of C/EBPα to bind to chromatin and thereby inhibits C/EBPα-induced transcription and neutrophil differentiation ( Fig. 8 ). 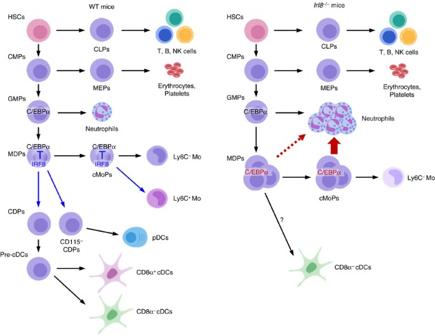Figure 8: Schematic representation of haematopoiesis in WT andIrf8−/−mice. WT MDPs and cMoPs express high levels of IRF8 protein. IRF8 binds to and inhibits the transcriptional activity of C/EBPα in these mononuclear phagocyte progenitors, thereby preventing C/EBPα-mediated neutrophil differentiation. InIrf8−/−mice, MDPs and cMoPs accumulate, and due to the derepression of C/EBPα activity,Irf8−/−MDPs and cMoPs give rise to massive numbers of neutrophils. IRF8 is also required for the development of Ly6C+monocytes, CDPs, pre-cDCs, CD8α+cDCs and pDCs. Figure 8: Schematic representation of haematopoiesis in WT and Irf8 −/− mice. WT MDPs and cMoPs express high levels of IRF8 protein. IRF8 binds to and inhibits the transcriptional activity of C/EBPα in these mononuclear phagocyte progenitors, thereby preventing C/EBPα-mediated neutrophil differentiation. In Irf8 −/− mice, MDPs and cMoPs accumulate, and due to the derepression of C/EBPα activity, Irf8 −/− MDPs and cMoPs give rise to massive numbers of neutrophils. IRF8 is also required for the development of Ly6C + monocytes, CDPs, pre-cDCs, CD8α + cDCs and pDCs. Full size image Our present data indicate that essentially all ‘CD115 + ’ MDPs and >80% of ‘ Cx3cr1 -GFP + ’ MDPs highly express IRF8, a finding which is somewhat distinct from the results of a recent study of transgenic mice harbouring a phage artificial chromosome (PAC) sequence containing three copies of the Irf8 gene fused to internal ribosome entry site (IRES)-YFP. In that study, ~50% of ‘ Cx3cr1 -GFP + ’ MDPs were found to express Irf8 via a PU.1-dependent mechanism [18] . We also note that while our present data indicate that LSK cells barely express IRF8, the above-mentioned study reported that all LSK cells already express Irf8 at even higher levels than MDPs. The reason for these discrepancies is unknown, but may be because the earlier report used the exogenous PAC sequence and monitored the transcription level of Irf8 . Whatever the reason for the discrepancies, our current results indicate that IRF8 protein expression sharply increases only when myeloid progenitor cells progress to MDPs. By comparing WT and Irf8 −/− mice, we have demonstrated herein that Irf8 −/− myeloid progenitors accumulate at the MDP and cMoP stages. Irf8 −/− mice lack CD117 low MDPs/CDPs, CD115 − CDPs, pre-cDC and Ly6C + monocytes that pinpoints the steps at which differentiation arrest occurs in these mice. Indeed, when transplanted, Irf8 −/− MDPs and cMoPs failed to efficiently give rise to DCs and monocytes. Scheller et al . [7] reported in 1999 through an in vitro colony-forming assay of bone marrow cells that Irf8 −/− colonies are mostly of a neutrophil morphology, even in the presence of M-CSF. We have also previously demonstrated that a significant fraction of Irf8 −/− Lin − cells respond to M-CSF to generate neutrophils [22] . These seemingly anomalous observations can now be explained by our present finding that MDPs and cMoPs, which are CD115 (M-CSF receptor)-expressing progenitor populations within Lin − cells, give rise to neutrophils in vivo if IRF8 is lost. We infer from this that the production of neutrophils derived from MDPs and cMoPs is a major cause of neutrophilia in Irf8 −/− mice because mononuclear phagocyte progenitors are the first populations at which IRF8 is highly expressed in the myeloid lineage, and MDPs and cMoPs accumulate in Irf8 −/− mice. Whether all Irf8 −/− MDPs pass through cMoPs to produce neutrophils is unknown; some Irf8 −/− MDPs may directly differentiate into neutrophils. Interestingly, Bhattacharya and colleagues [17] have recently reported that all lymphoid progenitors (ALPs) from Irf8 −/− mice can produce neutrophils. Therefore Irf8 −/− ALPs may also contribute to neutrophilia. Our transcriptome analysis of MDPs and cMoPs from WT and Irf8 −/− mice predicted that C/EBP(s) is aberrantly activated in the absence of IRF8. Indeed, C/EBPα binding to its target genes was significantly increased in these Irf8 −/− CD115 + progenitor cells. From the results of co-immunoprecipitations of exogenously expressed proteins, an AlphaScreen using recombinant proteins and PLA for endogenous proteins, we concluded that IRF8 directly interacts with C/EBPα, which is known to promote neutrophil differentiation, in MDPs and cMoPs. Domain analysis indicated that this interaction involves DBDs of IRF8 and C/EBPα. Consistent with these findings, IRF8 inhibits chromatin binding and transactivation activities of C/EBPα and thereby blocks C/EBPα-induced neutrophil differentiation. The ability of IRF8 to stimulate monocyte and DC differentiation is not a consequence of inhibiting C/EBPα activity and neutrophil differentiation, because the IRF8 R289E mutant can still do the latter but not the former, and the inhibition of C/EBP activity in Irf8 −/− haematopoietic progenitors selectively restored neutrophil overproduction. Interestingly, IRF8 did not reverse C/EBPα-induced growth arrest. This suggests the possibility that C/EBPα does not require its DNA binding activity to halt cell growth. Indeed, it has been reported previously that C/EBPα arrests cell proliferation by directly binding to E2F via the TE-I domain during adipogenesis and granulopoiesis [33] , and to Cdk2 and Cdk4 via the TE-III domain in the liver [37] . In support of such a notion, the introduction of C/EBPα significantly inhibited the expression of various known E2F target genes in 32Dcl.3 cells, and this inhibition was not affected by the coexpression of IRF8 ( Supplementary Fig. 8a ). Moreover, reporter assays in 32Dcl.3 cells transduced with a lentivirus carrying an E2F-responsive luciferase construct showed that IRF8 does not reverse the inhibitory effects of C/EBPα upon E2F transcriptional activity ( Supplementary Fig. 8b ). We note that in addition to the direct inhibition of C/EBPα activity by IRF8 via physical interaction, it is also possible that IRF8 induces the expression of genes encoding proteins that then inhibit chromatin binding of C/EBPα and/or neutrophil differentiation. Indeed, although the IRF8 R289E mutant, which can interact with C/EBPα but not with PU.1 or other IRFs, suppressed C/EBPα-mediated neutrophil differentiation, this inhibition was less potent than WT IRF8. Our finding that IRF8 inhibits chromatin binding of C/EBPα but not the other way around has implications for the interplay between three key myeloid transcription factors, IRF8, C/EBPα and PU.1, that have now all been found to interact with each other. Both C/EBPα-PU.1 (ref. 38 ) and C/EBPα–IRF8 interactions involve the DBDs of these three transcription factors. On the other hand, the IRF8–PU.1 interaction occurs between the IRF association domain and the PEST domain, respectively [39] . We infer from this that the binding affinity of the IRF8–PU.1 heterodimer for its target DNA element may be higher than that for its interaction with C/EBPα homodimer. This notion is supported by our two findings, that is, the chromatin binding of IRF8 is not inhibited by C/EBPα, and these two transcription factors do not colocalize on chromatin. This model also suggests that the expression level of IRF8 may need to be high enough to inhibit C/EBPα activity, as in MDPs and cMoPs. Because the DBDs of the C/EBP family are conserved and A-C/EBP can inhibit any C/EBP, the activity of C/EBPs other than C/EBPα might be also inhibited by IRF8. When overexpressed in 293T cells, IRF8 did bind to and inhibit transcriptional activation by C/EBPε, and IRF8 was found to inhibit the C/EBPε-mediated induction of target genes and neutrophil differentiation in 32Dcl.3 cells ( Supplementary Fig. 9 ). However, since Cebpe expression levels are low in cells highly expressing IRF8, the interaction between IRF8 and C/EBPε may not occur in vivo . Another possibility would be an involvement of C/EBPβ, which has been shown to be required for emergency granulopoiesis [40] . The inhibition of C/EBP by IRF8 may also operate in other cell lineages where both IRF8 and C/EBP are expressed. For example, IRF8 is expressed in pre-osteoclasts and inhibits their differentiation, whereas C/EBPα is expressed in both pre-osteoclasts and osteoclasts to promote osteoclastogenesis [41] , [42] . Moreover, because the DBDs are well conserved in both the IRF and C/EBP families, other IRF–C/EBP interactions may also occur. Adipocytes are a good candidate because they express multiple IRFs and C/EBPs, and IRF3 and IRF4 repress, while some C/EBPs stimulate, adipogenesis [43] , [44] . In conclusion, IRF8 was found to have a critical role in determining the differentiation characteristics of mononuclear phagocyte progenitor populations. IRF8 thus appears to have a dual role in stimulating and inhibiting cell differentiation within myeloid cell lineages by cooperating with other key transcription factors. Mice Male and female Ly5.1, Ly5.2, Irf8 −/− and Cx3cr1 gfp/+ mice [45] in a C57BL/6 background were used at 7–9 weeks of age. All animal experiments were conducted in accordance with the Guidelines for Proper Conduct of Animal Experiments (Science Council of Japan), and all protocols were approved by institutional review boards of Yokohama City University (protocol no. F11-85). Flow cytometry and separation of haematopoietic progenitors Splenocytes were isolated by liberase and DNase I (Roche) treatment. Bone marrow cells were harvested by flushing femurs and tibias. Flow cytometry was performed using a FACSCanto II (BD Biosciences), and data were analysed using FlowJo software (Tree Star). For staining lineage marker-positive cells, the Lineage Cell Detection Cocktail (biotinylated anti-CD5, CD45R (B220), CD11b, Gr-1 (Ly6G/C), Ter-119 and 7-4 antibodies; Miltenyi Biotec) was used. Other antibodies and their clone names were anti-CD117 (2B8), Sca-1 (D7), CD16/32 (93), CD115 (ASF98), Flt3 (A2F10), CD3 (145-2C11), CD11b (M1/70), CD19 (6D5), Ly6C (HK1.4), MHC-class II (AF6-120.1), CD11c (N418), CD8α (53-6.7), CD4 (GK1.5) and Ly6G (1A8) antibodies from Biolegend and anti-CD34 (RAM34) and NK1.1 (PK136) antibodies from eBioscience. Anti-IRF8 (C-19) and C/EBPα (AA14) antibodies for intracellular immunostaining were purchased from Santa Cruz Biotechnology. The antibodies used including dilutions are listed in Supplementary Table 1 . For staining surface makers, cells were incubated for 30 min at 4 °C with appropriately diluted fluorochrome-conjugated antibodies or biotinylated antibodies, and then with fluorochrome-conjugated streptavidin. 7-amino-actinomycin D (Sigma) was used to exclude dead cells. Intracellular staining of transcription factors was performed as described previously [14] . Briefly, cells were fixed with 4% paraformaldehyde, permeabilized with 0.5% saponin (Sigma-Aldrich), blocked with 10% normal donkey serum and stained with goat anti-IRF8, rabbit anti-C/EBPα antibody, control normal goat IgG or normal rabbit IgG (Jackson ImmunoResearch). This was followed by incubation with fluorochrome-conjugated donkey anti-goat or anti-rabbit antibody. For isolation of bone marrow MDPs (defined as Lin − IL-7R − Sca-1 − CD117 + CD115 + cells) [26] , [46] , Lin − cells were first enriched using the Lineage Cell Depletion Kit and magnetic-activated cell sorting (MACS) system (Miltenyi Biotec). For the isolation of cMoPs (defined as CD3 − CD11b − CD19 − Ly6G − NK1.1 − Flt3 − CD117 + CD115 + Ly6C + cells) [20] and CD115 + progenitor cells (defined as CD3 − CD11b − CD19 − Ly6G − NK1.1 − CD117 + CD115 + cells), bone marrow cells were first incubated with biotinylated anti-CD3, CD19, Ly6G and NK1.1 antibodies and then with anti-Biotin MicroBeads (Miltenyi Biotec), followed by negative selection. Enriched Lin − cells or CD3 − CD19 − Ly6G − NK1.1 − cells were then stained with appropriate antibodies and sorted using FACSAria II (BD Biosciences). The purity of the sorted cells was always >99%. Adoptive transfer and culture of bone marrow progenitors MDPs or cMoPs purified from Ly5.2 mice (CD45.2 + ) were injected intravenously into lethally irradiated (950 rad) Ly5.1 mice (CD45.2 − ; 1.0 × 10 4 cells per mouse). These mice were killed 5 and 2 days after the MDP and cMoP transfer, respectively, and the progeny cells in the bone marrow and spleen were analysed. For in vitro culture, sorted MDPs (5.0 × 10 3 cells ml −1 ) were treated with SCF (100 ng ml −1 ), M-CSF (20 ng ml −1 ), Flt3L (100 ng ml −1 ) and G-CSF (20 ng ml −1 ) in RPMI1640 medium (Nacalai Tesque) supplemented with 20% heat-inactivated fetal bovine serum. Harvested cells were counted and stained with anti-CD11b and Ly6G antibodies, followed by flow cytometric analyses. Microarray and IPA MDPs, cMoPs and 32Dcl.3 cells [10] were subjected to microarray analysis using the RNeasy Micro Kit (Qiagen), the Low Input Quick Amp Labeling Kit (Agilent), a Whole Mouse Genome 8 × 60K Microarray (Agilent) and an Agilent DNA Microarray Scanner, in accordance with the manufacturer’s protocols. All data were normalized using quantile methods and analysed by NIA Array Analysis software ( http://lgsun.grc.nia.nih.gov/ANOVA/ ). Visualization of hierarchical clustering and primary component analysis were also performed using the NIA Array Analysis software. P values were determined by one-way analysis of variance test. Among the microarray probes, only those associated with RefSeq or Ensembl protein-coding transcripts were selected for analysis. To predict transcription factors that could explain the upregulation of certain genes (FC >3 and FDR <0.05) in Irf8 −/− progenitors compared with WT progenitors, Ingenuity Upstream Regulator Analysis was performed using IPA software version 8.8 (Ingenuity Systems; www.ingenuity.com ). This analysis was based on compiled knowledge from the literature describing relationships between regulators and their target genes (Ingenuity Knowledge Base), and calculates a Z -score using a prediction algorithm ( http://pages.ingenuity.com/rs/ingenuity/images/0812%20upstream_regulator_analysis_whitepaper.pdf ). In accordance with the manufacturer’s instructions, Z -scores >2.0 were considered significant. All microarray data are available at the GEO/NCBI database (accession code GSE50052 ). Microarray data for HSCs have been previously published [47] . Reporter assay The pcDNA3.1-HA-C/EBPα vector was constructed by inserting a restriction enzyme site-tagged Cebpa cDNA obtained by PCR from a pMSV-C/EBPα plasmid into pcDNA3.1(+) (Invitrogen) in which a HA epitope (HA tag) had been inserted. pcDNA3.1-IRF8, pcDNA3.1-IRF8 K79E and pcDNA3.1-IRF8 R289E were constructed by the subcloning of cDNAs from pMSCV plasmids into pcDNA3.1(+). The C/EBP reporter lentiviral vector, pGreenFire1-C/EBPα-EF1-puro (System Biosciences) and two packaging vectors (pCMV-VSV-G and pCMVΔR8.2; RIKEN BioResource Center) were transiently transfected into HEK293T cells. After 48 h, the lentivirus-containing supernatants were harvested and used to transduce 293T cells, which were then selected by puromycin treatment at 2 μg ml −1 . The reporter 293T cells were transfected with pcDNA3.1-C/EBPα and/or pcDNA3.1-IRF8, pcDNA3.1-IRF8 K79E or pcDNA3.1-IRF8 R289E using Lipofectamine LTX (Invitrogen). Twenty-four hours after transfection, GFP expression was analysed by flow cytometry. For the E2F reporter assay, 32Dcl.3 cells were transduced with Cignal E2F Reporter lentivirus (Qiagen), and selected under puromycin at 2 μg ml −1 . The reporter 32Dcl.3 cells were transduced with empty MSCV-neo or MSCV-IRF8-neo vectors, and then with empty MSCV-CD8t or MSCV-C/EBPα-CD8t. Transduced cells were selected using 500 μg ml −1 G-418 (Roche) and MACS sorting. Two days after C/EBPα transduction, cells were lysed using the Dual-Glo Luciferase Assay System and analysed in a GloMax 96 Microplate Luminometer (Promega). Quantitative PCR with reverse transcription Total RNA was prepared using NucleoSpin RNA II (Macherey-Nagel) and reverse transcribed using the PrimeScript RT reagent kit (Takara) in accordance with the manufacturer’s instructions. The following primers were used in the RT–qPCR analyses: Csf3r (sense, 5′- TTGCCCACCATCATGACAGA -3′; antisense, 5′- GAATCCCAGTGGGTCGGTTT -3′), Elane (sense, 5′- TGACTAACATGTGCCGCCGT -3′; antisense, 5′- GAGTCCCCGAAGCAGATGCC -3′), Gfi1 (sense, 5′- ACAGGTGAGAAGCCCCACAA -3′; antisense, 5′- CCACACAGGTCACAGCCAAA -3′), Ltf (sense, 5′- TGTGCTCCCAACAGCAAAGA -3′; antisense, 5′- GCCTTCTCAGCCAGACACCTTA -3′), Aif1 (sense, 5′- CAGAATGATGCTGGGCAAGA -3′; antisense, 5′- GGACCAGTTGGCCTCTTGTG -3′), Irf5 (sense, 5′- ATGTCCTGGACCGTGGGCTC -3′; antisense, 5′- GAACACCTTACACTGGCACAGACG -3′), Ctss (sense, 5′- TGGCAAAGATTACTGGCTTGTG -3′; antisense, 5′- GCCATCCGAATGTATCCTTGA -3′) and Entpd1 (sense, 5′- GGGCAAGATCAAAGACAGCAA -3′; antisense, 5′- GTTCAGCTGGGATCATGTTGG -3′). Retroviral transduction The pMSCV-IRF8-CD8t construct that carries the Irf8 cDNA in pMSCV-CD8t (MSCV-IRES-human-truncated CD8; a kind gift from Dr Ricardo A. Feldman) has been described previously [15] , [48] . pMSCV-IRF8 K79E -CD8t and pMSCV-IRF8 R289E -CD8t were generated by subcloning of the cDNAs from pMSCV-IRF8 K79E -puro and pMSCV-IRF8 R289E -puro, respectively [10] . pMSCV-C/EBPα-puro was constructed by inserting restriction enzyme site-tagged Cebpa cDNA obtained by PCR from pMSV-C/EBPα [49] , a kind gift from Dr Alan D. Friedman, into pMSCV-puro (MSCV-PGK-puromycin resistant gene; Clontech). To construct pMSCV-C/EBPε-puro, restriction enzyme site-tagged Cebpe cDNA, obtained by RT–PCR from C/EBPα-transduced 32Dcl.3 cells, was inserted into pMSCV-puro. pGCsam-IRES-EGFP and pGCsam-A-C/EBP-IRES-EGFP vectors [35] were kindly provided by Dr Atsushi Iwama. For retroviral transduction [15] , 293T cells were transiently transfected with retroviral vectors and the pCL-Eco packaging vector using Lipofectamine 2000 (Life Technologies) in accordance with the manufacturer’s protocol. Retroviral supernatants were collected at 48 and 72 h. Cells were transduced by spinoculation (1,300 g , 30 °C, 90 min) in a retroviral supernatant supplemented with cytokines and 4 μg ml −1 polybrene. Transduced cells were selected by puromycin treatment (2 μg ml −1 ) or MACS sorting. Co-immunoprecipitation pcDNA3.1(+) plasmids carrying HA-tagged C/EBPα mutants, Δ11-70 (ΔTE-I), Δ70-97 (ΔTE-II) and Δ97-257 (ΔTE-III) were constructed by inserting restriction enzyme site-tagged cDNAs obtained by PCR from the pMSV-C/EBPαΔ1-2, pMSV-C/EBPαΔ3 and pMSV-C/EBPαΔ4-9 vectors, respectively, kindly provided by Dr Alan D. Friedman [49] into pcDNA3.1(+) with a HA tag. cDNAs encoding C/EBPαΔDBD, C/EBPαΔDBD+NLS from SV40 large T antigen, C/EBPαΔBR+NLS and C/EBPαΔLZ+NLS were generated by PCR using primers tagged with restriction enzyme sites (and the NLS sequence) and inserted into pcDNA3.1(+) with a HA tag. The pcDNA3.1-FLAG-C/EBPα vector was generated by subcloning the cDNA from pcDNA3.1-HA-C/EBPα into pcDNA3.1(+) in which a FLAG tag had been inserted. 293T cells were transfected with empty pcDNA3.1, pcDNA3.1-HA-C/EBPα (WT or its mutants) and/or pcDNA3.1-IRF8 (WT or its point mutants) using Lipofectamine LTX. Forty-eight hours after transfection, cells were lysed with lysis buffer (50 mM Tris-HCl, 300 mM NaCl, 2 mM EDTA and 1% Nonidet P-40). Protein G-coated Dynabeads (Invitrogen) were washed twice in lysis buffer, followed by incubation with a goat anti-IRF8 antibody (C-19; Santa Cruz Biotechnology). After washing in lysis buffer, the primary antibody-conjugated Protein G Dynabeads were incubated with cell lysates at 4 °C for 16 h with gentle shaking, followed by washing twice in lysis buffer. For FLAG-tagged C/EBPα immunoprecipitation, anti-FLAG M2 magnetic beads (Sigma-Aldrich) were added to the lysates and incubated at 4 °C for 16 h with gentle shaking, followed by five washes in lysis buffer. Immunoprecipitates were eluted with SDS sample buffer, boiled for 10 min, subjected to SDS–polyacrylamide gel electrophoresis and blotted with antibodies for IRF8 (C-19), C/EBPα antibody (14AA; Santa Cruz Biotechnology), HA (12CA5; Roche), β-actin (AC-15; Sigma-Aldrich) or FLAG (M2; Sigma-Aldrich). Uncropped scans of the western blots are shown in Supplementary Figs 10–12 . C/EBPα-YFP chimeric proteins The pEYFP-C1 vectors carrying C/EBPα and its mutants, Δ11-70 (ΔTE-I), Δ70-97 (ΔTE-II) and Δ97-257 (ΔTE-III) were constructed by inserting restriction enzyme site-tagged cDNAs obtained by PCR from pMSV-C/EBPα, pMSV-C/EBPαΔ1-2, pMSV-C/EBPαΔ3 and pMSV-C/EBPαΔ4-9, respectively, into pEYFP-C1 (Clontech). cDNAs encoding C/EBPαΔDBD and C/EBPαΔDBD+NLS were generated by PCR using primers tagged with restriction enzyme sites (and the NLS sequence) and inserted into pEYFP-C1. The pEYFP-C1 vectors carrying C/EBPαΔBR+NLS and C/EBPαΔLZ+NLS sequences were generated by subcloning the cDNA insert from pcDNA3.1-HA-C/EBPαΔBR+NLS and pcDNA3.1-HA-C/EBPαΔLZ+NLS, respectively, into pEYFP-C1. HeLa cells were transfected with pEYFP-C1-C/EBPα (WT or its mutants) and pHcRed-C1 (Clontech) using Lipofectamine LTX. Forty-eight hours after transfection, cells were stained with Hoechst 33342, followed by confocal microscopy. AlphaScreen The pEU-E01-IRF8-FLAG construct was generated by subcloning the cDNA from pMSCV-IRF8-FLAG-puro [15] . The pEU-E01 vector (Cell Free Science) is a plasmid vector specifically developed for the wheat-germ cell-free protein synthesis system [50] . pEU-E01-C/EBPα biotin-ligating sequence was constructed by inserting restriction enzyme site-tagged Cebpa cDNA obtained by PCR from pMSV-C/EBPα into pEU-E01 into which a biotin-ligating sequence had been inserted. These plasmids were then used as templates for in vitro protein synthesis using the wheat-germ expression kit (CellFree Science). FLAG-tagged IRF8 proteins were mixed with biotinylated C/EBPα in 15 μl of reaction buffer (20 mM Tris-HCl, pH 7.6, 5 mM MgCl 2 and 1 mM dithiothreitol in a well of 384-well optiplates (PerkinElmer) and incubated at 26 °C for 1 h. The mixture was then added to AlphaScreen buffer containing anti-immunoglobulin G (protein A) acceptor beads, streptavidin-coated donor beads (PerkinElmer) and the anti-FLAG M2 antibody (Sigma), and further incubated at 26 °C. One hour later, AlphaScreen signals from the mixture were detected using an EnVision device (PerkinElmer) with the AlphaScreen signal detection program. In situ PLA Purified MDPs and cMoPs were fixed by 4% paraformaldehyde and cytospun on Matsunami adhesive silane (MAS)-coated glass slides. Cells were then permeabilized in 100% methanol and PLA was performed using Duolink in situ PLA (OLINK Biosciences) in accordance with the manufacturer’s instructions. As primary antibodies, goat anti-IRF8 (C-19) and rabbit anti-C/EBPα (2295; Cell Signaling Technology) antibodies were used. For negative control experiments, normal goat IgG and normal rabbit IgG (Santa Cruz Biotechnology) were used. The secondary antibodies used were anti-goat (for IRF8) and anti-rabbit (for C/EBPα) antibodies conjugated to complementary synthetic oligonucleotides. PLA signals were visualized by confocal microscopy (FV1000-D; Olympus). ChIP–qPCR ChIP–qPCR assays were performed as described previously [9] , except that cells were fixed with 1% formaldehyde for 10 min at room temperature and the reaction was quenched with 125 mM glycine. The lysates were sonicated 20 times for 1 min each with a Bioruptor sonicator (Cosmo Bio). Immunoprecipitation was then performed using Dynabeads Protein G (Veritas) coated with a goat anti-IRF8 antibody (C-19), a rabbit anti-C/EBPα antibody (14AA), control normal goat IgG or normal rabbit IgG. The following primers were used in the qPCR analysis: Aif1 (sense, 5′- CTTTCCACTCATTCCCTTGCTAACT -3′; antisense, 5′- TCAGCACATTACTTCTTCATCTCCTC -3′), Ltf (sense, 5′- TTAGCCAACTGTGTGTTTCTTCACA -3′; antisense, 5′- AGGGTCCCTCATTTGGAAACAATA -3′), Ctss (sense, 5′- CAACATGGAGCAAGCCAGTG -3′; antisense, 5′- CTTCCGGAACATTCCACACC -3′), Entpd1 (sense, 5′- CCCCCAGCTAGTACTCACCA -3′; antisense, 5′- GTGGGCTGACTCCAGGATAA -3′), Elane (sense, 5′- TGCTGACATGGAGACCCTGA -3′; antisense, 5′- ACCAGAGGCCGTTGTATTGC -3′), Csf3r (sense, 5′- TTTCCCTCAACCTCCTTCCTG -3′; antisense, 5′- CCAGAATTGCGACACCTTCC -3′), Hsd11b1 (sense, 5′- GTAAATGTTCCAACACTCCCACTTC -3′; antisense, 5′- GCTGCTTTTATAGAGGAAAGCTTGG -3′), S100a8 (sense, 5′- GTAAATGTTCCAACACTCCCACTTC -3′; antisense, 5′- GCTGCTTTTATAGAGGAAAGCTTGG -3′), Cebpe (sense, 5′- GGATCTTGCAACACTGGGATG -3′; antisense, 5′- AGGTGAGTCTACCAAGGTCAGTCAG -3′), and Klf4 (sense, 5′- AGACGAGATTAAGCTAAAGGGGACA -3′; antisense, 5′- AGAGTAGTTGAGCTCTTGCTGTTGG -3′). C/EBPα binding sites on the Cebpe gene were predicted from previously published ChIP followed by deep sequencing (ChIP-seq) data for histone H3 lysine 27 acetylation and histone H3 lysine 4 monomethylation in bone marrow cells [51] . Adoptive transfer of retrovirus-transduced progenitor cells Lin − cells isolated from WT or Irf8 −/− bone marrow were cultured with interleukin (IL)-6 (10 ng ml −1 ), SCF (100 ng ml −1 ) and IL-3 (10 ng ml −1 ) in RPMI1640 supplemented with 20% heat-inactivated fetal bovine serum for 24 h, and then transduced with retroviral vectors (GCsam-IRES-EGFP or GCsam-A-C/EBP-IRES-EGFP) by spinoculation. Four hours after transduction, cells were washed and transplanted into irradiated (950 rad) WT mice. Three weeks after transplantation, splenocytes were isolated by liberase and DNase I treatment and analysed by flow cytometry. How to cite this article: Kurotaki, D. et al . IRF8 inhibits C/EBPα activity to restrain mononuclear phagocyte progenitors from differentiating into neutrophils. Nat. Commun. 5:4978 doi: 10.1038/ncomms5978 (2014). Accession codes: Microarray data have been deposited in the NCBI Gene Expression Omnibus under accession code GSE50052 .